P-Rex1 is required for efficient melanoblast migration and melanoma metastasis Metastases are the major cause of death from melanoma, a skin cancer that has the fastest rising incidence of any malignancy in the Western world. Molecular pathways that drive melanoblast migration in development are believed to underpin the movement and ultimately the metastasis of melanoma. Here we show that mice lacking P-Rex1, a Rac-specific Rho GTPase guanine nucleotide exchange factor, have a melanoblast migration defect during development evidenced by a white belly. Moreover, these P-Rex1 −/− mice are resistant to metastasis when crossed to a murine model of melanoma. Mechanistically, this is associated with P-Rex1 driving invasion in a Rac-dependent manner. P-Rex1 is elevated in the majority of human melanoma cell lines and tumour tissue. We conclude that P-Rex1 has an important role in melanoblast migration and cancer progression to metastasis in mice and humans. Melanoma is an aggressive skin cancer characterized by its resistance to chemotherapy. Its incidence has doubled over the past two decades in the Western world. Patients who have primary melanomas with a Breslow thickness >4 mm have a dramatically increased incidence of metastasis and reduced survival [1] . Progression to melanoma is driven primarily by oncogenic mutations of BRAF (50–60%) or NRAS (15–30%) [2] , [3] , [4] , but must be accompanied by further genetic and epigenetic changes in gene expression, most commonly the loss of tumour suppressors p16INK4A or PTEN [5] , [6] . Present treatments with conventional chemotherapies have had no impact on overall survival, with the Braf V600E -targeted therapy, vemurafenib (PLX4032), recently giving cause for encouragement [7] , [8] . However, there remains a deficit of effective treatment strategies for other melanoma types, while treatment resistance to vemurafenib has been reported in melanomas coexpressing Nras Q61K with oncogenic Braf V600E (refs 9 and 10 ). PREX1 encodes the P-Rex1 Dbl family of Rho GTPase guanine nucleotide exchange factors (GEFs). Rho family small GTPases comprise a major branch of the Ras superfamily of small GTPases (for example, RhoA, Rac1 and Cdc42) [11] . P-Rex1 is a Rac-specific GEF stimulated by PI3K-stimulated phosphatidylinositol (3,4,5)-trisphosphate production and the β-gamma subunits of the heterotrimeric-G proteins (Gβγ), both of which bind to P-Rex1 (refs 12 , 13 , 14 ). It has also been identified as a transcriptional target of extracellular signal-regulated kinase (ERK) signalling across a panel of melanoma cell lines [15] . Rac, the main effector of P-Rex1 activity, is involved in the induction of actin-mediated membrane ruffling and lamellipodia formation at the leading edge of cell migration, and its aberrant activation has been implicated in tumour cell invasion and metastasis [16] , [17] . P-Rex1 has not previously been characterized in genetically modified animal models of cancer that can genetically and pathologically recapitulate the human disease. Earlier studies using cancer cell lines have implicated a role in prostate, breast and ovarian cancer [18] , [19] , [20] , [21] . Here we demonstrate that P-Rex1 is necessary for migration of melanoblasts during mouse development, it facilitates metastasis formation in an Nras Q61K -driven mouse model of melanoma, and it is upregulated in human melanoma-derived cell lines and tissue. P-Rex1-deficient mice have a white belly phenotype We first investigated the in vivo relevance of P-Rex1 by further analyses of a P-Rex1 −/− mouse [22] . We identified a 'white belly' phenotype with 100% penetrance in P-Rex1 −/− mice on a pure C57BL6 background ( Fig. 1a ). The phenotype persisted when P-Rex1 −/− mice were crossed with Tyr ∷ Nras Q61K/ ° transgenic mice ( Tyr ∷ Nras Q61K/ ° ; P-Rex1 −/− ), a major driver mutation in melanoma ( Fig. 1a ) [23] . Depigmentation affecting the feet was also observed in Tyr ∷ Nras Q61K/ ° ; P-Rex1 −/− mice ( Fig. 1a ). Tissue sections of bellies from P-Rex1 −/− and Tyr ∷ Nras Q61K/ ° ; P-Rex1 −/− mice suggested that no melanocytes were present throughout the skin in the white belly area ( Fig. 1b ). Thus expression of Nras Q61K was not able to overcome the 'white belly' induced by ablation of PREX1 . 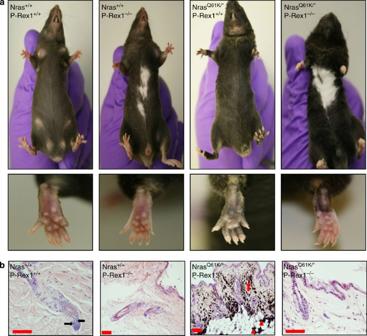Figure 1: P-Rex1-deficient mice have a 'white belly' phenotype. (a) Belly and feet of P-Rex1+/+and P-Rex1−/−mice in combination with both Nras+/+and NrasQ61K/°transgenic modification. (b) Photomicrographs (haematoxylin and eosin) of belly skin from the four genotypes represented in (a). Normal melanocyte situation in a C57BL6 mouse is in the hair follicles (black arrows). Melanocytes and deposition of melanin in the dermis (red arrow) and adipose tissue (red arrowheads) are seen in NrasQ61K/°mice. Scale bar, 100 μm. Figure 1: P-Rex1-deficient mice have a 'white belly' phenotype. ( a ) Belly and feet of P-Rex1 +/+ and P-Rex1 −/− mice in combination with both Nras +/+ and Nras Q61K/° transgenic modification. ( b ) Photomicrographs (haematoxylin and eosin) of belly skin from the four genotypes represented in ( a ). Normal melanocyte situation in a C57BL6 mouse is in the hair follicles (black arrows). Melanocytes and deposition of melanin in the dermis (red arrow) and adipose tissue (red arrowheads) are seen in Nras Q61K/° mice. Scale bar, 100 μm. Full size image P-Rex1 deficiency impairs normal melanoblast migration The belly, feet and tail are the furthermost points of mouse melanoblast migration from the neural crest during embryogenesis. In line with this and the role of P-Rex1 in activation of Rac, we hypothesized that the areas of depigmentation in P-Rex1 −/− mice predominantly represented a defect of melanoblast migration during embryogenesis, rather than an impaired proliferative capacity or inability to produce melanin pigment in adult melanocytes. To test this hypothesis, we first ensured the presence of PREX1 in melanoblasts ( Fig. 2a ). 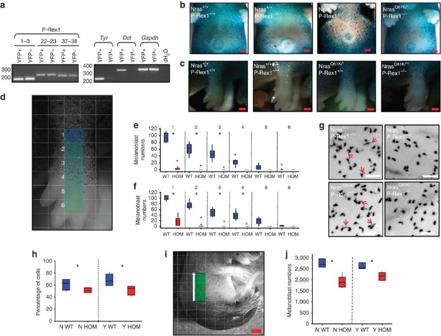Figure 2: P-Rex1−/−mice have a defect in melanoblast migration. (a) RT–PCR of P-Rex1 mRNA in E14.5 embryo skin following FACS selection of cells enriched for melanoblasts (yellow fluorescent protein, YFP+) compared with the rest of the embryo skin (YFP−). Tyrosinase and Dct controls confirm melanoblast enrichment. (b) E15.5 representative pictures comparing melanoblast migration to the belly in 5-bromo-4-chloro-3-indolyl-β-d-galactoside (X-gal)-stained embryos. Scale bars, 500 μm. (c) Comparison of melanoblast migration along the forepaw in X-gal-stained embryos at E15.5. A migratory deficit is evident in both P-Rex1−/−(with either Nras+/+or NrasQ61K/°) embryos. Scale bars, 500 μm. (d) Schematic picture detailing quantification of melanoblast migration in the forepaw at E15.5. Levels 1 to 6 from top to bottom represent areas of 500×500 μm. Melanoblasts counted at each level and numbers compared between genotypes. (e,f) Comparison of melanoblast migration between P-Rex1+/+(blue bars) and P-Rex1−/−(red bars) mice at levels 1 to 6 (as detailed ind). Upper panel (e) represents Nras+/+embryos (*P=0.01/0.02, levels 2/3; Mann–Whitney test,n=5), lower panel (f) represents NrasQ61K/°embryos (*P=0.02/0.02/0.01, levels 1/2/3; Mann–Whitney test,n=5; all box and whiskers plots: boxes represent 25th–75th percentiles of given value, lines represent median values). (g) Representative pictures at E15.5 of melanoblast morphology and protrusions (red arrows) on the flank of X-gal-stained embryos. Scale bars, 100 μm. (h) Quantification and comparison of percentage of cells with 1+ protrusions: P-Rex1+/+(N WT, blue bars) and P-Rex1−/−mice (N HOM, red bars; left-hand panel; *P=0.05, Mann–Whitney;n=4); and Tyr∷NrasQ61K/°; P-Rex1+/+(Y WT, blue bars) and Tyr∷NrasQ61K/°; P-Rex1−/−(Y HOM, red bars) mice (right-hand panel; *P=0.03; Mann–Whitney,n=4). (i) Schematic picture detailing quantification of melanoblast cell numbers at E15.5. Areas represented: 1×3 mm. (j) Comparison of E15.5 melanoblast numbers between P-Rex1+/+(N WT, blue bars) and P-Rex1−/−(N HOM, red bars) mice (left-hand panel), and also between Tyr∷NrasQ61K/°; P-Rex1+/+(Y WT, blue bars) and Tyr∷NrasQ61K/°; P-Rex1−/−(Y HOM, red bars) mice (right-hand panel) (left panel: *P=0.01; right panel: *P=0.01; Mann–Whitney test,n=5). Gapdh, glyceraldehyde-3-phosphate dehydrogenase; WT, wild type. Figure 2: P-Rex1 −/− mice have a defect in melanoblast migration. ( a ) RT–PCR of P-Rex1 mRNA in E14.5 embryo skin following FACS selection of cells enriched for melanoblasts (yellow fluorescent protein, YFP+) compared with the rest of the embryo skin (YFP−). Tyrosinase and Dct controls confirm melanoblast enrichment. ( b ) E15.5 representative pictures comparing melanoblast migration to the belly in 5-bromo-4-chloro-3-indolyl-β-d-galactoside (X-gal)-stained embryos. Scale bars, 500 μm. ( c ) Comparison of melanoblast migration along the forepaw in X-gal-stained embryos at E15.5. A migratory deficit is evident in both P-Rex1 −/− (with either Nras +/+ or Nras Q61K/° ) embryos. Scale bars, 500 μm. ( d ) Schematic picture detailing quantification of melanoblast migration in the forepaw at E15.5. Levels 1 to 6 from top to bottom represent areas of 500×500 μm. Melanoblasts counted at each level and numbers compared between genotypes. ( e , f ) Comparison of melanoblast migration between P-Rex1 +/+ (blue bars) and P-Rex1 −/− (red bars) mice at levels 1 to 6 (as detailed in d ). Upper panel ( e ) represents Nras +/+ embryos (* P =0.01/0.02, levels 2/3; Mann–Whitney test, n =5), lower panel ( f ) represents Nras Q61K/° embryos (* P =0.02/0.02/0.01, levels 1/2/3; Mann–Whitney test, n =5; all box and whiskers plots: boxes represent 25th–75th percentiles of given value, lines represent median values). ( g ) Representative pictures at E15.5 of melanoblast morphology and protrusions (red arrows) on the flank of X-gal-stained embryos. Scale bars, 100 μm. ( h ) Quantification and comparison of percentage of cells with 1+ protrusions: P-Rex1 +/+ (N WT, blue bars) and P-Rex1 −/− mice (N HOM, red bars; left-hand panel; * P =0.05, Mann–Whitney; n =4); and Tyr ∷ Nras Q61K/° ; P-Rex1 +/+ (Y WT, blue bars) and Tyr ∷ Nras Q61K/° ; P-Rex1 −/− (Y HOM, red bars) mice (right-hand panel; * P =0.03; Mann–Whitney, n =4). ( i ) Schematic picture detailing quantification of melanoblast cell numbers at E15.5. Areas represented: 1×3 mm. ( j ) Comparison of E15.5 melanoblast numbers between P-Rex1 +/+ (N WT, blue bars) and P-Rex1 −/− (N HOM, red bars) mice (left-hand panel), and also between Tyr ∷ Nras Q61K/° ; P-Rex1 +/+ (Y WT, blue bars) and Tyr ∷ Nras Q61K/° ; P-Rex1 −/− (Y HOM, red bars) mice (right-hand panel) (left panel: * P =0.01; right panel: * P =0.01; Mann–Whitney test, n =5). Gapdh, glyceraldehyde-3-phosphate dehydrogenase; WT, wild type. Full size image To address whether melanoblast number or migratory behaviour was altered, we next analysed P-Rex1 −/− and Tyr ∷ Nras Q61K/ ° ; P-Rex1 −/− mice that had been intercrossed with mice carrying the DCT-lacZ transgene, a melanoblast reporter line [24] . Melanoblast sparing of the feet and belly was apparent in both DCT-lacZ P-Rex1 −/− and DCT-lacZ Tyr ∷ Nras Q61K/ ° ; P-Rex1 −/− mice at E15.5, excluding a defect in melanin production as a cause for their depigmentation ( Fig. 2b,c ). Using a melanoblast migration assay, which compared differences in distal melanoblast migration at various points of development ( Fig. 2d ; Supplementary Fig. S1a ), analysis of E13.5 and E15.5 embryos showed a statistical difference in melanoblast migration between DCT-lacZ P-Rex1 −/− and DCT-lacZ P-Rex1 +/+ mice ( Fig. 2e ; Supplementary Fig. S1b ). This was not overcome by Nras Q61K/ ° expression ( Fig. 2f ; Supplementary Fig. S1b ). Consistent with a migratory defect, melanoblasts on the flank of the DCT-lacZ P-Rex1 −/− mice had fewer protrusions than DCT-lacZ P-Rex1 +/+ controls ( Fig. 2g,h ). A melanoblast cell number assay at E13.5 showed no difference in cell numbers between DCT-lacZ P-Rex1 −/− and DCT-lacZ P-Rex1 +/+ mice unless DCT-lacZ P-Rex1 −/− mice were intercrossed with Tyr ∷ Nras Q61K/ ° mice ( Supplementary Figs S2a,b ). There was however a small but significant reduction of E15.5 cell numbers in DCT-lacZ P-Rex1 −/− mice compared with DCT-lacZ P-Rex1 +/+ , and DCT-lacZ Tyr ∷ Nras Q61K/ ° ; P-Rex1 −/− compared with DCT-lacZ Tyr ∷ Nras Q61K/ ° ; P-Rex1 +/+ mice ( Fig. 2i,j ). This difference is likely to represent a proliferative deficit in P-Rex1 −/− melanoblasts: cell death was not observed in E15.5 whole skin from P-Rex1 +/+ or P-Rex1 −/− mouse embryos, using a live ex vivo imaging technique that we have previously described ( Supplementary Movies 1 , 2 , 3 ) [25] . Moreover, a significant reduction in E15.5 cell numbers was again seen in P-Rex1 −/− embryos compared with P-Rex1 +/+ controls using this technique ( Supplementary Fig. S2c ). Collectively, these results would be consistent with previous reports of a role for Rac in cell cycle control, as well as the proliferative defect observed when P-Rex1 was knocked down in breast cancer cell lines [21] , [26] , [27] . They suggest that a small proliferative defect is preceded by a marked migration defect in P-Rex1 −/− mice. P-Rex1 deficiency impairs metastasis in a melanoma mouse model The imprint of past migratory behaviour of neural crest–derived melanocyte precursors has been suggested to confer a propensity of primary melanomas to establish distant metastases [28] , [29] , [30] . We therefore crossed P-Rex1 −/− mice with a genetically modified model of metastatic malignant melanoma, Tyr ∷ Nras Q61K/ ° ; INK4a −/− mice, to assess whether P-Rex1 may also be important for primary melanoma development and/or metastasis [23] . Tyr ∷ Nras Q61K/ ° ; INK4a −/− ; P-Rex1 +/+ mice developed primary melanoma and metastasis with a similar penetrance and latency to that previously described ( Fig. 3a ). Immunohistochemistry (IHC) was carried out on primary melanomas taken from P-Rex1 +/+ and P-Rex1 −/− mice to confirm P-Rex1 expression in tumours ( Fig. 3b,c ). Seven out of ten primary melanomas from P-Rex1 +/+ mice showed staining for P-Rex1, compared with zero out of nine samples from P-Rex1 −/− mice. All metastases from P-Rex1 +/+ mice displayed immunoreactivity for P-Rex1 similar to that of MelanA (11 samples; lung, liver and brain; Fig. 3d ). 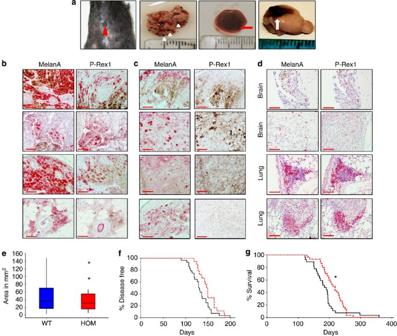Figure 3: P-Rex1−/−mice have significantly reduced metastases in a Tyr∷NrasQ61K/°; INK4a−/−murine melanoma model. (a) Primary and metastatic melanomas arising in Tyr∷NrasQ61K/°; INK4a−/−transgenic mice. Red arrowhead: pigmented primary skin melanoma; white arrowheads: multiple pigmented lung metastases; red arrow: pigmented liver metastasis; white arrow: large pigmented brain lesion. (b) MelanA and P-Rex1 immunohistochemical expression in primary melanomas of P-Rex1+/+mice. Varying levels of P-Rex1 expression can be seen in mouse melanomas (pink staining)n=10. (c) MelanA and P-Rex1 immunohistochemical expression in primary melanomas of P-Rex1−/−mice. No P-Rex1 expression was observed in melanomas from these micen=9. (d) MelanA and P-Rex1 immunohistochemical expression in melanoma metastases from P-Rex1+/+control mice. Upper four panels show expression in brain lesions, while lower four panels show expression in lung metastases (pink staining)n=11. (e) Comparison of primary tumour burden between Tyr∷NrasQ61K/°; INK4a−/−; P-Rex1+/+(blue bar) and Tyr∷NrasQ61K/°; INK4a−/−; P-Rex1−/−(red bar) mice (P=0.43, Mann–Whitney,n=29; small asterisks represent outlying data; box and whiskers plot: box represent 25th–75th percentile of given value, line represents median value). (f) Kaplan–Meier analysis of primary melanoma latency between Tyr∷NrasQ61K/°; INK4a−/−; P-Rex1+/+(black line,n=27) and Tyr∷NrasQ61K/°; INK4a−/−; P-Rex1−/−(red line,n=18) cohorts (P=0.156, log-rank test). (g) Kaplan–Meier curves detailing significant improvement in survival of Tyr∷NrasQ61K/°; INK4a−/−; P-Rex1−/−cohort (red line) compared with Tyr∷NrasQ61K/°; INK4a−/−; P-Rex1+/+cohort (black line; *P=0.017, log-rank test,n=30 for each cohort). WT, wild type. Figure 3: P-Rex1 −/− mice have significantly reduced metastases in a Tyr ∷ Nras Q61K/° ; INK4a −/− murine melanoma model. ( a ) Primary and metastatic melanomas arising in Tyr ∷ Nras Q61K/° ; INK4a −/− transgenic mice. Red arrowhead: pigmented primary skin melanoma; white arrowheads: multiple pigmented lung metastases; red arrow: pigmented liver metastasis; white arrow: large pigmented brain lesion. ( b ) MelanA and P-Rex1 immunohistochemical expression in primary melanomas of P-Rex1 +/+ mice. Varying levels of P-Rex1 expression can be seen in mouse melanomas (pink staining) n =10. ( c ) MelanA and P-Rex1 immunohistochemical expression in primary melanomas of P-Rex1 −/− mice. No P-Rex1 expression was observed in melanomas from these mice n =9. ( d ) MelanA and P-Rex1 immunohistochemical expression in melanoma metastases from P-Rex1 +/+ control mice. Upper four panels show expression in brain lesions, while lower four panels show expression in lung metastases (pink staining) n =11. ( e ) Comparison of primary tumour burden between Tyr ∷ Nras Q61K/° ; INK4a −/− ; P-Rex1 +/+ (blue bar) and Tyr ∷ Nras Q61K/° ; INK4a −/− ; P-Rex1 −/− (red bar) mice ( P =0.43, Mann–Whitney, n =29; small asterisks represent outlying data; box and whiskers plot: box represent 25th–75th percentile of given value, line represents median value). ( f ) Kaplan–Meier analysis of primary melanoma latency between Tyr ∷ Nras Q61K/° ; INK4a −/− ; P-Rex1 +/+ (black line, n =27) and Tyr ∷ Nras Q61K/° ; INK4a −/− ; P-Rex1 −/− (red line, n =18) cohorts ( P =0.156, log-rank test). ( g ) Kaplan–Meier curves detailing significant improvement in survival of Tyr ∷ Nras Q61K/° ; INK4a −/− ; P-Rex1 −/− cohort (red line) compared with Tyr ∷ Nras Q61K/° ; INK4a −/− ; P-Rex1 +/+ cohort (black line; * P =0.017, log-rank test, n =30 for each cohort). WT, wild type. Full size image Although Rac function has been shown to be required for primary squamous cell skin and lung tumour development [31] , [32] , we observed no difference in incidence, latency or tumour burden of primary melanomas between Tyr ∷ Nras Q61K/ ° ; INK4a −/− ; P-Rex1 +/+ and Tyr ∷ Nras Q61K/ ° ; INK4a −/− ; P-Rex1 −/− mice ( Table 1 ; Fig. 3e,f ). However, a significant reduction in melanoma metastasis was observed in the Tyr ∷ Nras Q61K/ ° ; INK4a −/− ; P-Rex1 −/− cohort, with the number of metastases in control Tyr ∷ Nras Q61K/ ° ; INK4a −/− ; P-Rex1 +/+ mice the same as previously reported ( P =0.001; χ 2 -test; Table 1 ). Tyr ∷ Nras Q61K/o ; INK4a −/− ; P-Rex1 −/− mice also had an improved overall survival ( Fig. 3g ). These data are consistent with the mouse melanoblast data, suggesting that P-Rex1 is a central component of migration and invasion. Table 1 P-Rex1 −/− dramatically reduces incidence of metastasis in an Tyr ∷ Nras Q61K/° ; INK4a −/− transgenic murine melanoma model. Full size table Although we are unable to categorically exclude the possibility that our melanoma brain lesions are not primary melanocytic neoplasms of the central nervous system (CNS), a significant reduction in metastases was still seen when these lesions were excluded from our analysis ( Table 1 ). Clearly they at least invade the brain parenchyma from either a blood-borne metastasis or the lepto-meningeal site of origin in primary CNS melanoma ( Fig. 3d ). In support of them being genuine metastases, no Nras Q61K mutations were observed in a previous study of human primary CNS melanoma [33] . We next further explored the prometastatic role of endogenous P-Rex1 in melanoma by deriving melanocyte cell lines from the early pup skin of Tyr ∷ Nras Q61K/ ° ; INK4a −/− ; P-Rex +/+ and Tyr ∷ Nras Q61K/ ° ; INK4a −/− ; P-Rex1 −/− mice. When injected via tail vein (TV) into C57BL6 mice, two out of four mice treated with Tyr ∷ Nras Q61K/ ° ; INK4a −/− ; P-Rex1 −/− melanocytes were found to have metastases, compared with five out of five mice who were treated with Tyr ∷ Nras Q61K/ ° ; INK4a −/− ; P-Rex +/+ cells ( Supplementary Table S1 , Supplementary Fig. S3 ). A significant reduction in metastatic frequency was observed on histological analyses of the cohort injected with Tyr ∷ Nras Q61K/ ° ; INK4a −/− ; P-Rex1 −/− melanocytes, with a clear reduction in metastatic tumour burden also seen ( Supplementary Fig. S3a,b ). Moreover, we observed a propensity of the Tyr ∷ Nras Q61K/ ° ; INK4a −/− ; P-Rex +/+ cells to metastasize to distant viscera (kidney, liver, heart and spleen), metastases that were not seen in the mice TV-treated with Tyr ∷ Nras Q61K/ ° ; INK4a −/− ; P-Rex1 −/− cells ( Supplementary Table S1, Supplementary Fig. S3c–g ). Collectively, these results suggested that endogenous P-Rex1 can facilitate frequency, growth and organ spread of metastases in melanoma from the intravasation stage of the metastatic cascade. These data in genetically modified models of cancer were also supported by analyses of immuno-deficient mice which were injected subcutaneously with a number of different human melanoma-derived cell lines ( Supplementary Fig. S4a,b, Supplementary Table S2 ). In total, 17/24 cell lines developed tumours following injection, with 4/24 also forming metastases. Quantitative reverse transcription (RT)–PCR ( Supplementary Methods ) analysis revealed that, of the cell lines with P-Rex1 mRNA levels above the median ('high' P-Rex1), nearly all went on to develop tumours in immuno-deficient mice ( Supplementary Figs. S4a ). This included all mice that developed metastases, and notably, the two Nras Q61K and Braf V600E cell lines with the highest P-Rex1 mRNA levels both developed metastases. Statistical evaluation of these results confirmed that high P-Rex1 was 100% statistically sensitive for detecting those nude mice that developed metastases ( Supplementary Table S3 ; P =0.005; χ 2 -test). P-Rex1 levels were highest in cell lines that form metastases after averaging P-Rex1 levels in cell lines that formed no tumours, tumours or metastases ( Supplementary Fig. S4b ). The lowest expression occurred in those cell lines that do not form tumours in immuno-deficient mice ( Supplementary Fig. S4b ). P-Rex1 is upregulated and drives invasion in human melanoma To test the relevance of our data to human melanomagenesis, we first examined the expression of P-Rex1 in established human melanoma cell lines derived from primary or metastatic disease. Compared with normal human melanocytes (NHM), there was marked P-Rex1 overexpression in nearly all of the cell lines ( Fig. 4a ). Moreover, the three cell lines with clearly the highest P-Rex1 expression (CHL1, SK-Mel119 and Mel224) were all derived from a metastatic source ( Supplementary Table S4 ), supporting our above analysis that showed high P-Rex1 mRNA was sensitive for the development of metastases in TV-treated immuno-deficient mice ( Supplementary Fig. S4 ). 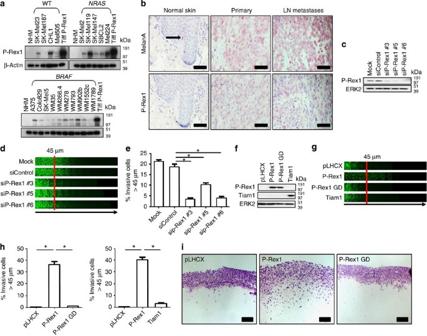Figure 4: P-Rex1 is upregulated in human melanoma where it drives invasion through its RacGEF activity. (a) Western blots illustrating endogenous expression of P-Rex1 in a panel of human melanoma-derived cell lines. Cell lines with driver mutations inNRASandBRAFare represented, along with cell lines that are WT for both. NHM, normal human melanocytes. (b) P-Rex1 expression increases with more aggressive disease. Photomicrographs of human tissue specimens of normal skin, primary and metastatic melanoma, immunohistochemically labelled against P-Rex1 or the melanocyte marker melanA. LN, lymph node. Scale bars, 90 μm. (c) Silencing P-Rex1 by siRNA as shown by western blot analysis. A mock transfection and scramble siRNA were used as controls. (d) Comparison of representative matrigel invasion assays of CHL1 human melanoma cell lines treated with control or P-Rex1-specific siRNA oligonucleotides. (e) Quantification of cells invading beyond 45 μm in matrigel invasion assays of CHL1 human melanoma cell lines treated with control ('siControl') versus P-Rex1 ('siP-Rex1')-specific siRNA oligonucleotides (*P=0.005, Mann–Whitney test;n=3; error bars, ±s.e.m). (f) Western blot confirming relative expression of 'P-Rex1', 'P-Rex1 GD' and 'Tiam1' cells is well matched. (g) Representative matrigel invasion assays comparing melanocytes derived from early pup skin ofTyr∷NrasQ61K/°; INK4a−/−; P-Rex1−/−mice, genetically modified to overexpress P-Rex1 ('P-Rex1'), empty vector ('pLHCX'), GEF-dead P-Rex1 ('P-Rex1 GD') or Tiam1 ('Tiam1'). (h) Left panel: quantification of cells invading beyond 45 μm in matrigel invasion assays of pLHCX versus P-Rex1 versus P-Rex1 GD cells (*P⩽0.0001 for both comparisons, Mann–Whitney test;n=3). Right panel: quantification of cells invading beyond 45 μm in matrigel invasion assays of pLHCX versus P-Rex1 versus Tiam1 cells (*P⩽0.0001 for both comparisons, Mann–Whitney test;n=3; error bars for both panels, ±s.e.m.). (i) Representative organotypic invasion assays comparingTyr∷NrasQ61K/°; INK4a−/−; P-Rex1−/−parental melanocytes genetically manipulated to overexpresswild-typeP-Rex1 ('P-Rex1'), empty vector ('pLHCX') and 'P-Rex1 GD' (n=3; scale bars, 90 μm). WT, wild type. Figure 4: P-Rex1 is upregulated in human melanoma where it drives invasion through its RacGEF activity. ( a ) Western blots illustrating endogenous expression of P-Rex1 in a panel of human melanoma-derived cell lines. Cell lines with driver mutations in NRAS and BRAF are represented, along with cell lines that are WT for both. NHM, normal human melanocytes. ( b ) P-Rex1 expression increases with more aggressive disease. Photomicrographs of human tissue specimens of normal skin, primary and metastatic melanoma, immunohistochemically labelled against P-Rex1 or the melanocyte marker melanA. LN, lymph node. Scale bars, 90 μm. ( c ) Silencing P-Rex1 by siRNA as shown by western blot analysis. A mock transfection and scramble siRNA were used as controls. ( d ) Comparison of representative matrigel invasion assays of CHL1 human melanoma cell lines treated with control or P-Rex1-specific siRNA oligonucleotides. ( e ) Quantification of cells invading beyond 45 μm in matrigel invasion assays of CHL1 human melanoma cell lines treated with control ('siControl') versus P-Rex1 ('siP-Rex1')-specific siRNA oligonucleotides (* P =0.005, Mann–Whitney test; n =3; error bars, ±s.e.m). ( f ) Western blot confirming relative expression of 'P-Rex1', 'P-Rex1 GD' and 'Tiam1' cells is well matched. ( g ) Representative matrigel invasion assays comparing melanocytes derived from early pup skin of Tyr ∷ Nras Q61K/ ° ; INK4a −/− ; P-Rex1 −/− mice, genetically modified to overexpress P-Rex1 ('P-Rex1'), empty vector ('pLHCX'), GEF-dead P-Rex1 ('P-Rex1 GD') or Tiam1 ('Tiam1'). ( h ) Left panel: quantification of cells invading beyond 45 μm in matrigel invasion assays of pLHCX versus P-Rex1 versus P-Rex1 GD cells (* P ⩽ 0.0001 for both comparisons, Mann–Whitney test; n =3). Right panel: quantification of cells invading beyond 45 μm in matrigel invasion assays of pLHCX versus P-Rex1 versus Tiam1 cells (* P ⩽ 0.0001 for both comparisons, Mann–Whitney test; n =3; error bars for both panels, ±s.e.m.). ( i ) Representative organotypic invasion assays comparing Tyr ∷ Nras Q61K/ ° ; INK4a −/− ; P-Rex1 −/− parental melanocytes genetically manipulated to overexpress wild-type P-Rex1 ('P-Rex1'), empty vector ('pLHCX') and 'P-Rex1 GD' ( n =3; scale bars, 90 μm). WT, wild type. Full size image We next assessed whether increased P-Rex1 activity in humans is also related to melanoma progression: this possibility was raised by both the sensitivity of high P-Rex1 mRNA for nude mouse metastasis development and the increased expression of P-Rex1 observed in melanoma-derived cell lines compared with normal melanocytes. IHC for P-Rex1 was performed on human tissue specimens from skin and melanoma: although P-Rex1 expression was not detectable in melanocytes in normal skin (3 out of 3 specimens), we consistently detected it in biopsies of primary melanomas (112 out of 141 specimens) and melanoma lymph node metastases (8 out of 9 specimens; Fig. 4b ; Supplementary Fig. S5 ). These data provided further evidence of a role for P-Rex1 in human melanoma progression, and were consistent with our previous findings in mice. One potential way that P-Rex1 could drive progression and metastatic spread is through an increased invasive capacity conferred by its RacGEF activity. To examine this, we knocked down endogenous P-Rex1 in the CHL1 human melanoma cell line, where P-Rex1 was upregulated ( Fig. 4a) . Consistently we observed that three-dimensional (3D) matrigel invasion was diminished following knockdown of endogenous P-Rex1 ( Fig. 4c–e ). This result was also reproducible in the WM793 human melanoma cell line used in our RT–PCR data ( Supplementary Fig. S6a–c ). As P-Rex1 is overexpressed in the majority of human melanoma cell lines, we used the previously described melanocyte cell line derived from early pup skin of Tyr ∷ Nras Q61K/ ° ; INK4a −/− ; P-Rex1 −/− mice to examine invasion in a cell line where P-Rex1 is not endogenously expressed. These P-Rex1 −/− cell lines, which were genetically manipulated to overexpress empty vector ('pLHCX'), failed to invade in 3D matrigel and organotypic assays unless they were re-constituted to express ectopic levels of P-Rex1 ('P-Rex1'; Fig. 4f–i ). Expression of ectopic levels of GEF-dead P-Rex1 ('P-Rex1 GD') failed to phenocopy the invasive phenotype of cells with re-constituted wild-type P-Rex1, confirming the RacGEF activity of P-Rex1 as a downstream mechanism ( Fig. 4f–i ). Interestingly, ectopic expression of another RacGEF described in melanoma, TIAM1, also failed to phenocopy the invasion seen with P-Rex1 expression ( Fig. 4f–h ) [34] . These results showed that the RacGEF activity of P-Rex1 may have a unique role among RacGEFs: it functions as a vital component of invasion for cells of the melanocyte lineage, a mechanism by which it can drive melanoma progression and metastases. Here we evaluated the role of a Rac-specific Rho GTPase GEF, P-Rex1, for the first time in a genetically modified animal model of cancer. In particular, we have examined its role in melanoma progression, invasion and metastasis. First, we showed that P-Rex1 has a role in progression with our human cell line and IHC analysis showing P-Rex1 upregulation in tumour compared with NHMs. Second, matrigel and organotypic invasion assays confirmed that P-Rex1 is a key component of invasion in both humans and mice, channelled through its RacGEF activity. Finally and most importantly, we have determined that genetic ablation of PREX1 impairs melanoma metastases in Tyr ∷ Nras Q61K ; INK4a −/− mice. Taken together, these results confirm that P-Rex1 upregulation is an important component of melanoma progression, invasion and metastatic signalling, supporting the value of pharmacological inhibition of P-Rex1 activation of Rac for treatment of metastatic or high-risk primary melanomas. Mechanistic experiments in our study have highlighted the key similarities between the molecular machinery involved in the movement of melanoblasts and that of metastatic melanoma cells. Genetic ablation of PREX1 impaired migration of melanoblasts, evidenced by a 'white belly' phenotype that reflected the diminished metastases seen in Tyr ∷ Nras Q61K ; INK4a −/− mice. A potential pathophysiological link with incidence of metastases therefore fits the physiological role of P-Rex1 seen in melanoblast migration. Moreover, the predominant role of P-Rex1 in invasion and migration is reflected by its presence in motile melanoblasts and its upregulation in metastatic melanoma cell lines. Other studies have previously suggested a role for P-Rex1 in prostate, breast and ovarian cancer [18] , [19] , [20] , [21] , with key similarities existing between our study and that of Sosa et al . [19] in particular. Notably, this report identified P-Rex1 as having particular relevance to the specific ER+ (+/− ErbB2) subset of breast tumours. One key area to focus on next will be to assess whether the in vivo tumourigenic effects of P-Rex1 are specific to melanomas driven by oncogenic Nras, or reproducible in Braf V600E -driven tumours: this is a clear possibility given the identification of P-Rex1 as a transcriptional target of ERK signalling in melanoma [15] . These previous P-Rex1 cancer studies have also shown an effect on both primary tumour growth and lymph node metastases using xenotransplantation of human cancer cell lines into immuno-deficient mice. However, this technique often fails to recapitulate the characteristics of the original tumour they are meant to represent, and their use for informative studies of novel cancer target validation has become increasingly contentious [35] , [36] , [37] . A key advance in our study is therefore the characterization of P-Rex1 in animal models of cancer, which recapitulate the common human genetics of the disease. Strategies for inhibiting RAS have long been a therapeutic challenge [9] . Our findings suggest that targeting P-Rex1 signalling might have great relevance to tumours driven or codriven by oncogenic RAS , with potential benefits extending to all melanomas [10] . There is limited but growing evidence that Rho GTPase guanine nucleotide exchange factors are tractable targets for the development of small-molecule inhibitors [17] . The lack of P-Rex1 expression in most other normal human cell types offers a clear therapeutic window and basis for selective cytotoxicity [14] , [37] . Here we have identified P-Rex1 as a novel anticancer target in melanoma. Our experiments provide stringent preclinical validation of P-Rex1 in cancer using informative genetically defined mouse models that recapitulate common human mutations. Together with recent observations in other cancers [18] , [19] , [20] , [21] , we suggest that P-Rex1 is an important therapeutic target for the treatment of a diverse spectrum of human cancers. Embryo analysis and β-galactosidase staining All studies were conducted in accordance with UK home office guidelines. Time of gestation was calculated using noon on the day of detection of a vaginal plug as E0.5, but also noting and comparing the external appearance of the embryo. Embryos were dissected at E15.5 then fixed in 0.25% glutaraldehyde at 4 °C for 45 min on a rolling platform. Embryos washed in PBS at 4 °C for 15 min on a rolling platform, detergent washed (2 mM MgCl 2 , 0.01% Na-deoxycholate, 0.02% NP-40 in PBS) at room temperature three times (30 min, 15 min two times). β-Galactosidase substrate (1 M MgCl 2 , 0.02% NP-40, 0.01% Na-deoxycholate, 0.04% 5-bromo-4-chloro-3-indolyl-β- D -galactoside, 5 mM K 3 Fe(CN) 6 , 5 mM K 4 Fe(CN) 6 ) was then added to the embryos, which were incubated in darkness overnight. Embryos were postfixed in 4% paraformaldehyde for 2 h at 4 °C. For cell number assays, the area used for quantification of cell numbers represented the most proximal point of melanoblast migration from the neural crest which could be accurately assayed. Counting melanoblasts in more distal regions would have introduced a migrational component to the assay which we aimed to avoid. Mouse treatment and survival cohorts A total of 80 Tyr ∷ Nras Q61K/° ; INK4a −/− and 10 C57BL6 mice were monitored for up to 18 months for the development of melanoma and signs of metastasis. All mice were checked thrice weekly for the development of malignant melanoma or any other pathology. End point criteria were melanomas ≥15 mm, ulcerating melanomas, cachexia, significant weight loss, or weakness and inactivity. Upon meeting these criteria, mice were euthanized. Mice were examined for the presence of frank metastasis upon dissection, but also visualization of haematoxylin-and-eosin (H&E)-stained sections for further identification of microscopic metastases. Organs/tumours were removed and fixed in 10% buffered formalin overnight at room temperature. Fixed tissues were paraffin embedded, and 5 mm sections were placed on sialynated/poly- L -lysine slides for immunohistochemical analysis. Lymph node metastases were not included in this analysis due to difficulty in distinguishing them from normal melanocyte populations that can be found in lymphoid tissue. For TV-injections into C57BL6 mice, cultured cells were maintained in antibiotic-free media for 1 week before injection. Cells were detached with trypsin, then blocked through suspension in complete culture media supplemented with 10% fetal bovine serum (FCS). Cells subjected to two rounds of washing, involving centrifugation at 100 g for 5 min followed by resuspension in 1× Hanks' Balanced Salt Solution (HBSS). Cells were finally resuspended in HBSS to a concentration of 1×10 7 cells ml −1 and TV injected at 1×10 6 cells per animal in a volume of 100 μl. Immunohistochemistry For P-Rex1, serial sections were unmasked in 10 mM citric acid, pH 6.0, with boiling for 30 min. Remaining steps were carried out with Thermo ScientificUltraVision LP Detection System (Thermo Fischer Scientific). Primary antibody was incubated in the presence of 5% normal goat serum (Dako). Antigens were developed with Vector Red Alkaline Phosphatase Substrate Kit (Vector Labs). The following antibody dilutions were used: P-Rex1, 1:100; MelanA, 1:100. 'Positive' staining refers to any level of staining visualized. Antibodies Rabbit polyclonal raised against human P-Rex1 (HPA001927) and mouse monoclonal specific to β-actin (clone AC-15, A1978) were obtained from Sigma-Aldrich. Mouse monoclonal specific to Melan-A (clones DT101 + BC199, ab731) was obtained from Abcam Ltd. Human tissues A tissue microarray was performed on archival paraffin patient samples from St Vincent's University Hospital, Dublin, Ireland. Quadruplicate cores from 141 consecutive melanoma patients (1994–2007) were used to construct the tissue microarray. Further samples were received from Radboud University Medical Center, Nijmegen, the Netherlands. All patient specimens were used in accordance with institutional and national policies at the respective locations. Statistical analyses Statistical analyses in mice were carried out using Minitab version 15 for Windows. Cell migration, invasion and cell number differences were determined using Mann–Whitney test. Distinction of metastasis and primary melanoma incidence was achieved using χ 2 -testing. Survival differences were determined with log-rank testing. All P -values were considered significant at P ⩽ 0.05. All appropriate value sets were tested for normality using a Kolmogorov–Smirnoff normality test. Cell culture NHMs were maintained in Mln254 medium (M-254-500, Cascade Biologics) supplemented with human melanocyte growth serum (S-002-5, Cascade Biologics) and penicillin/streptomycin at 100 U ml −1 . Mel224, Mel505, SK-Mel 2, 5, 23, 119, 147 and 187, CHL-1, A375 and WM266.4 were maintained in Dulbecco's modified Eagle medium supplemented with 10% FCS, L -glutamine at 200 μM and penicillin/streptomycin at 100 U ml −1 . SBCL2, Lu1205, WM852, MeWo, Dauv-1, Gerlach, 888mel, 501mel, MNT-1, WM 35, 278, 793, 902b, 1552c and 1789 were maintained in RPMI 1640 supplemented with 10% FCS and penicillin/streptomycin at 100 U ml −1 . For melanocyte isolation from mice, pup skin was dissected at P2 then placed in ice-cold PBS. Quickly it was cut into pieces and incubated in 1.5 ml of collagenase types 1 and 2 at 37 °C, 5% CO 2 for approximately 25–50 min. Contents transferred into 10 ml wash buffer (1× HBSS, 1 mM CaCl 2 , 0.005% DNase) and centrifuged at 200 g for 5 min at room temperature. Sample resuspended in 2 ml dissociation buffer, placed in small Petri dish and incubated at 37 °C, 5% CO 2 for 10 min. Thereafter, sample was put through an 18G then 20G needle and transferred into 10 ml wash buffer for 10 min. Supernatant centrifuged at 200 g for 5 min at room temp, pellet resuspended in 2 ml PBS, then re-centrifuged at 200 g for 5 min. Resuspended and maintained in RPMI 1640 medium supplemented with 10% FCS, L -glutamine at 200 μM and penicillin/streptomycin at 100 U ml −1 . siRNA treatments and RacGEF constructs Stable cell lines expressing Myc-epitope tagged human P-Rex1 were generated by retroviral infection using the modified Retro-X retroviral expression system (Clontech). An Hpa I restriction site, followed by Kozak consensus translation initiation site was introduced to the 5′ end of the coding sequence of myc-P-Rex1 (ref. 13 ), myc-P-Rex1 GEF-dead [13] or myc-Tiam1 by PCR (5′-GTTAACCACCATGGAGCAGAAGCTGATC-3′), with a Cla I restriction site introduced to the 3′ end in the same reaction (P-Rex1/P-Rex1 GEF-dead: 5′-CCATCGATTCAGAGGTCCCCATCCACCGG-3′), with pCMV-P-Rex1, pCMV-P-Rex1 GEF-dead or pcDNA3.1-myc-Tiam1 used as template. In each case, the Hpa I– Cla I DNA fragments produced were subcloned into Hpa I and Cla I sites of the pLHCX retroviral expression vector. High-titre, replication-incompetent retroviral particles encoding the RNA of interest were produced in the Phoenix Ampho packaging line (Orbigen), for human target cells, and the Phoenix Eco packaging line (Orbigen) for murine target cells. Subsequent infection of target lines resulted in transfer of the coding region of interest, along with a selectable marker. Pooled cell lines stably expressing the construct of interest were isolated by selection with hygromycin-B (500 μg ml −1 ) over multiple passages. Control lines were infected with retroviral particles expressing an empty pLHCX control vector transcript, and subjected to an identical selection procedure. Expression of the ectopically introduced proteins of interest was determined by western blot and immunodetection with both epitope-tag-specific and protein-specific primary antibodies. Transient knockdown of target proteins was achieved through consecutive rounds of liposome-mediated transfection with the appropriate small interfering RNA (siRNA) oligonucleotides, 48 h apart. Liposomal transfection reagent (301702, HiPerFect), non-targeting control oligonucleotides (1027281, AllStars Negative Control) and P-Rex1-specific oligonucleotides (SI00692405, Hs_PREX1_3; SI03144449, Hs_PREX1_5; SI03246383, Hs_PREX1_6) were obtained from Qiagen Ltd. Invasion assays For inverted Matrigel invasion assays [38] , Matrigel protein matrix (BD Bioscience) was allowed to polymerize in Transwell permeable inserts (Corning Ltd) over a period of 60 min at 37 °C. Inserts were inverted, and cells seeded directly onto the filter surface in complete growth medium. Cells were then allowed to adhere over a period of 3 h at 37 °C, after which both non-adherent cells and residual growth medium were removed with three washes in appropriate serum-free medium. Finally, inserts were placed in serum-free tissue culture medium (containing 10% FCS) above the Matrigel matrix to function as a chemoattractant. In the case of siRNA-mediated transient knockdown experiments, invasion assays were prepared 24 h after the second round of lipofection. At 72-h postseeding, invasive cells that had entered Matrigel were stained with the fluorescent live-cell dye Calcein-AM, and visualized through confocal microscopy of optical sections obtained in the z-plane at 15 μm intervals. Quantification was with the Area Calculator plugin for ImageJ ( http://rsbweb.nih.gov/ij/ ). For organotypic invasion assays [39] , approximately 7.5×10 4 ml −1 primary human fibroblasts were embedded in a 3D matrix of rat tail collagen I. Rat tail tendon collagen solution was prepared by the extraction of tendons with 0.5 M acetic acid to a concentration of ∼ 2 mg ml −1 . Detached, polymerized matrix (2.5 ml) in 35-mm Petri dishes was allowed to contract for approximately 6 days in complete media (DMEM, supplemented with 10% FCS; Invitrogen) until the fibroblasts had contracted the matrix to ∼ 1.5 cm diameter. Subsequently, Tyr ∷ Nras Q61K/ ° ; INK4a −/− ; P-Rex1 −/− melanocytes, stably expressing either control vector, human P-Rex1 or a GEF-dead mutant of human P-Rex1, were seeded onto the prepared matrix in complete media (4×10 4 cells per assay) and allowed to grow to confluence for 5 days. The matrix was then mounted on a metal grid and raised to the air/liquid interface resulting in the matrix being fed from below with complete media that was changed every 2 days. After 15 days, the cultures were fixed with 4% paraformaldehyde and processed by standard methods for haematoxylin and eosin staining. How to cite this article: C. R. Lindsay et al . P-Rex1 is required for efficient melanoblast migration and melanoma metastasis. Nat. Commun. 2:555 doi: 10.1038/ncomms1560 (2011).